miRNomes of haematopoietic stem cells and dendritic cells identify miR-30b as a regulator of Notch1 Dendritic cells (DCs) are critical to initiate the immune response and maintain tolerance, depending on different status and subsets. The expression profiles of microRNAs (miRNAs) in various DC subsets and haematopoietic stem cells (HSCs), which generate DCs, remain to be fully identified. Here we examine miRNomes of mouse bone marrow HSCs, immature DCs, mature DCs and IL-10/NO-producing regulatory DCs by deep sequencing. We identify numerous stage-specific miRNAs and histone modification in HSCs and DCs at different differentiation stages. miR-30b, significantly upregulated via a TGF-beta/Smad3-mediated epigenetic pathway in regulatory DCs, can target Notch1 to promote IL-10 and NO production, suggesting that miR-30b is a negative regulator of immune response. We also identify miRNomes of in vivo counterparts of mature DCs and regulatory DCs and systematically compare them with DCs cultured in vitro . These results provide a resource for studying roles of miRNAs in stem cell biology, development and functional regulation of DC subsets. Dendritic cells (DCs), the most potent professional antigen-presenting cells, are crucial for the initiation of innate and adaptive immune responses and also important in maintaining immune tolerance to self-tissues [1] . Together with all blood cells, DCs have their ultimate origin in haematopoietic stem cells (HSCs). HSCs have the capacity to self-renew over the lifespan and also to give rise to a series of precursor cells that are progressively committed to particular cell lineages [2] . Which precursor type will actually generate DCs will depend on the availability of precursors and the immune microenvironment involved [3] . In most circumstances, myeloid precursors are the main sources to generate DCs. DCs comprise a network of subsets that differ in location, migratory pathways, detailed immunological function and dependence on stimuli for their generation, adding further layers of complexity in the coordination of immune responses [4] . The developmental pathways that lead HSCs to the different DC subsets are very important, not just in the initial establishment of the DC network, but as dynamic components of the response to microbial invasion and the maintenance of immune homeostasis [5] . Although the development and differentiation pathways have been simply mapped and much knowledge has been gained about the origins, phenotypes and functions of mouse DC subsets, examining the mechanisms of gene regulation that underlie development from HSCs to different DC subsets has the potential to improve our understanding of cell differentiation in general and to provide insights for the development of clinically relevant DC-based immunotherapy. MicroRNAs (miRNAs) are an abundant class of evolutionarily conserved small non-coding RNAs that post-transcriptionally control gene expression by targeting mRNAs for degradation or translational repression, and have diverse functional roles in biological processes [6] . The endogenously expressed miRNAs have been identified as important contributors to many physiological and pathological processes including immune development and response [7] . It has been proven that miRNAs play an indispensable role in immune responses via regulating the development of monocytes/macrophages, DCs, NK cells, T cells and B cells, and also in regulating their responses to pathogens and stimulation with TLR ligands [8] , [9] , [10] , [11] , [12] , [13] . Although the contributions of few individual miRNAs to the development or function of HSCs and DCs have been reported, so far, the roles of miRNAs in the development and differentiation of DCs remain largely unknown. In adult mice, HSCs are originally described as precursors to all different subpopulations of DCs in the bone marrow. Upon inflammatory stimulation or uptake of pathogenic antigens, immature DCs (imDCs) undergo maturation and differentiate into mature DCs (maDCs), which are originally considered to be terminally differentiated [14] . However, our previous study demonstrated that splenic stromal cells, which mimic the secondary lymph organ microenvironment, can drive maDCs to further differentiate into regulatory DCs (DCreg) [15] . Therefore, the process of DC development and differentiation is very interesting, as it includes one development process (HSCs–imDCs), one maturation process (imDCs–maDCs) and one differentiation process (maDCs–DCreg), thus providing a good cell model to investigate how miRNAs are involved in different processes of cell differentiation and functional regulation. Up to now, a few studies have investigated this topic [16] , [17] , [18] , [19] ; however, a comprehensive profile of miRNAs in mouse bone marrow-derived DCs at different differentiation stages remain largely unknown. Massively parallel signature sequencing (MPSS) of miRNAs is a powerful approach to identify miRNome in-depth, and may reveal miRNA expression differences as well as the individual miRNA abundance in a given biological context, especially in the specific type of tissue or cell with definite differential or functional stage. Besides revealing the expression profile of known miRNAs, vast amounts of sequencing data enable exploration of novel miRNA [20] . To obtain a comprehensive quantitative expression profile of miRNAs in mouse bone marrow-derived DCs at different differentiation stages, in this study we establish miRNomes in bone marrow HSCs, imDCs, maDCs ( in vitro and in vivo ) and DCreg ( in vitro and in vivo ) using next-generation sequencing on Illumina platform. We demonstrate that about 391 miRNAs are differentially expressed during DC differentiation, with numerous stage-specific miRNAs regulated by histone modifications at different stages. A total of 121 miRNAs have the same alteration pattern during DC differentiation process (maDCs-DCreg) in vitro and in vivo . miR-30b, significantly upregulated in DCreg both in vitro and in vivo , is found to promote IL-10 and NO production through targeting Notch1. In addition, we reveal 53 new miRNA candidates. Our results may present a resource for researching the roles of miRNAs in the development and differentiation of DCs and also stem cell biology. miRNomes in mouse HSCs and DC subsets Using unique perfectly mapped reads, a total of 5,865,224, 5,928,841, 6,324,361 and 3,983,460 reads were sequenced from the HSCs, imDCs, maDCs and DCreg libraries respectively. We assigned each of the small RNAs a unique annotation according to its precursor and classified these small RNAs into different categories such as known miRNA, rRNA and so on (rRNA, tRNA, snRNA, snoRNA), repeat (LINE, SINE, LTR), mRNA (exons/introns) and unannotated small RNAs. All libraries showed a similar small RNA distribution. On average, 90.92% matched annotated miRNA hairpins; 7.06% matched rRNA, and so on. ; 1.35% matched mRNAs; 0.33% matched repeat elements and 0.34% were previously uncharacterized small RNAs ( Fig. 1a ). The mapping and categorizing of clean reads revealed that most small RNA reads were miRNAs during DC development and differentiation. 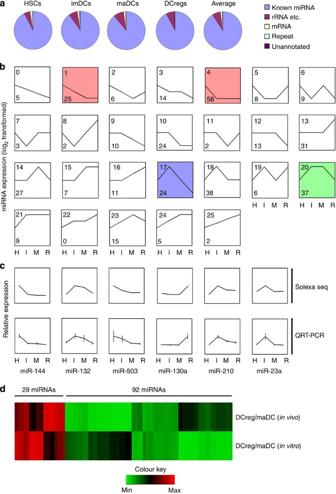Figure 1: Clustering of 391 differentially expressed miRNAs during DC development and differentiation. (a) Each small RNA sequence was assigned with a unique annotation and classified small RNAs into different categories such as known miRNA, rRNA and so on (rRNA, tRNA, snRNA, snoRNA), repeat (LINE, SINE, LTR), mRNA (exons/introns) and unannotated small RNAs. (b) The trend of 391 miRNAs was generally divided into 26 clusters according to their dynamic expression patterns among the four cell stages. Numbers on top left corner indicate the cluster number. Number on down left corner indicated the number of miRNAs in each cluster. The coloured clusters indicated significantly enriched ones by miRNAs (cluster 4 (red)P=0.0015; cluster 20 (green)P=0.0005; cluster 1 (red)P<0.00001; cluster 17 (blue)P=0.0001) (Fisher exact test). Three other expressions were normalized to the highest one in four stages firstly, and then all expressions were log2-transformed. (c) Six miRNAs were tested by qRT–PCR and compared with the results from Illumina sequencing. Three other expressions were normalized to the highest one in four stages firstly, and then all expressions were log2-transformed. (d) A total of 121 miRNAs with the same alteration pattern in process (maDCs-DCreg)in vitroandin vivowere selected. Expression of variation (fold) of each miRNAs between DCreg and maDCs was log-transformed and hierarchically clustered. H, HSCs; I, imDCs; M, maDCs; R, DCreg. Figure 1: Clustering of 391 differentially expressed miRNAs during DC development and differentiation. ( a ) Each small RNA sequence was assigned with a unique annotation and classified small RNAs into different categories such as known miRNA, rRNA and so on (rRNA, tRNA, snRNA, snoRNA), repeat (LINE, SINE, LTR), mRNA (exons/introns) and unannotated small RNAs. ( b ) The trend of 391 miRNAs was generally divided into 26 clusters according to their dynamic expression patterns among the four cell stages. Numbers on top left corner indicate the cluster number. Number on down left corner indicated the number of miRNAs in each cluster. The coloured clusters indicated significantly enriched ones by miRNAs (cluster 4 (red) P =0.0015; cluster 20 (green) P =0.0005; cluster 1 (red) P <0.00001; cluster 17 (blue) P =0.0001) (Fisher exact test). Three other expressions were normalized to the highest one in four stages firstly, and then all expressions were log2-transformed. ( c ) Six miRNAs were tested by qRT–PCR and compared with the results from Illumina sequencing. Three other expressions were normalized to the highest one in four stages firstly, and then all expressions were log2-transformed. ( d ) A total of 121 miRNAs with the same alteration pattern in process (maDCs-DCreg) in vitro and in vivo were selected. Expression of variation (fold) of each miRNAs between DCreg and maDCs was log-transformed and hierarchically clustered. H, HSCs; I, imDCs; M, maDCs; R, DCreg. Full size image miRNAs are differentially expressed at different DC stages In order to obtain the abundance value for each miRNA in each small RNA library, miRNAs in mouse miRBase v.19 were analysed and normalized to ‘transcripts per million (TPM)’ for each library. In order to depict the dynamic expression patterns of markedly changed miRNAs during DC development and differentiation, 391 miRNAs (TPM>10 in at least one small RNA library, acounting for ~99.9% of miRNome) were selected. The miRNA with more than double of expression variation between two analysed cell types was determined as differentially expressed miRNA. We further classified these miRNAs into the 26 possible dynamic expression patterns and calculated the number of miRNAs in each pattern. Fisher exact test was used to determine the significantly enriched patterns ( Fig. 1b ). Analysis showed that most miRNAs were expressed preferentially at one or two stages of DCs, and only a few of them were highly expressed in all the stages of DCs, suggesting miRNAs with specific functions may be more related to the biological characteristics of different DC stages. Tissue-specific expression of several miRNAs at certain stages of mammalian development has been reported [6] , [21] . As shown in Fig. 1a , miRNAs in cluster 4 were expressed highly in the HSCs, and these included some previously reported miRNAs such as miR-196b and miR-126 (refs 22 , 23 ), which is enriched in HSCs. miRNAs in cluster 13 were mainly expressed in DCregs, including miR-93 and let-7, which were reported to play important roles in regulating translation of differentiation-related key genes [24] . Cluster 0 was a very interesting cluster, these miRNAs gradually reduced in the commitment of HSCs to DCreg, suggesting that target genes of these continuously downregulated miRNAs participated in the development and differentiation of DCs. All miRNAs in each cluster were listed in Supplementary Data 1 . To validate the expression profiles obtained from Illumina sequencing, 32 miRNAs with different expression levels were tested by quantitative real-time RT–PCR (qRT–PCR). In all, 28 of 32 tested miRNAs (87.5%) correlated with the expression as detected by Illumina sequencing ( Supplementary Table S1 ). Six representative miRNAs that were correlated with the expression detected by Illumina sequencing were shown in Fig. 1c . To mutually corroborate the expression profiles obtained from in vitro DCs, CD11c + Ia high cells (the in vivo counterpart of mature DCs), CD11c + Ia low cells (the in vivo counterpart of regulatory DCs) from the murine splenocytes were sorted as described previously [15] . The total RNA was isolated and sequenced on Illumina platform. A total of 255 miRNAs (TPM>10 in at least one small RNA library) were selected for further analysis. We analysed the expression profile alteration in mature DCs—regulatory DCs development in vitro and in vivo . About half of miRNAs (121/255, 47.5%) have the same alteration pattern. Among these miRNAs, 29 miRNAs such as miR-30b, let-7, miR-146a and miR-22 increased their expression, whereas 92 miRNAs such as miR-132, miR-126, miR-93 and miR-146b decreased their expression in this process both in vivo and in vitro ( Fig. 1d ). So many miRNAs have same alteration pattern in vitro and in vivo , suggesting their specific biological functions in the process (maDCs-DCreg). All 255 miRNAs were listed in Supplementary Data 2 . Dynamic miRNA patterns at different DC stages Through Illumina sequencing, we first compared the variation of miRNA spectrums expressed in DCs during these processes, and found no obvious difference ( Fig. 2a ), as most of miRNA genes were co-expressed in these processes. Second, we analysed the expression variation of the 391 miRNAs in these processes. Through Pearson correlation scatter plot analysis, we found that there was no significant difference in expression levels of these miRNAs in the maturation process (imDCs–maDCs) ( r =0.921, Pearson’s correlation), whereas the difference was more obviously in the development process (HSCs–imDCs) ( r =0.767, Pearson’s correlation) and the differentiation process (maDCs–DCreg) ( r =0.893, Pearson’s correlation) ( Fig. 2b ). Similar results were also obtained from the differentiation process (maDCs–DCreg) in vivo ; most of the miRNA genes were co-expressed in this in vivo process ( Fig. 2c ) and significant difference in expression level was found ( r =0.891, Pearson’s correlation) ( Fig. 2d ). 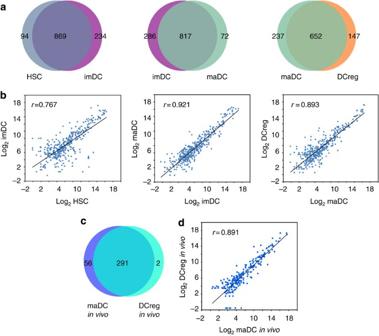Figure 2: miRNA profiles during DC development and differentiation. (a) Special and shared miRNAs in one development process (HSCs-imDCs), one maturation process (imDCs-maDCs) and one differentiation process (maDCs-DCreg). (b) Log base 2 intensity plots of miRNA levels in representative stages during DC development and differentiation. Pearson Correlationrvalues establish the linear fit of data. (c) Number and overlap of miRNAs in differentiation process (maDCs-DCreg)in vivo. (d) Log base 2 intensity plots of miRNA levels in differentiation process (maDCs-DCreg)in vivo. Pearson Correlationrvalues establish the linear fit of data. Figure 2: miRNA profiles during DC development and differentiation. ( a ) Special and shared miRNAs in one development process (HSCs-imDCs), one maturation process (imDCs-maDCs) and one differentiation process (maDCs-DCreg). ( b ) Log base 2 intensity plots of miRNA levels in representative stages during DC development and differentiation. Pearson Correlation r values establish the linear fit of data. ( c ) Number and overlap of miRNAs in differentiation process (maDCs-DCreg) in vivo . ( d ) Log base 2 intensity plots of miRNA levels in differentiation process (maDCs-DCreg) in vivo . Pearson Correlation r values establish the linear fit of data. Full size image From the above results, the variation of miRNA expression profile was significant in development and differentiation processes, but the alteration in maturation process was less significant. Stage-specific miRNAs undergo epigenetic reprogramming Although many miRNA promoters had been identified by using either a computational or experimental approach, numerous miRNA promoters still remain unclear. This difficulty persecuted the researches of epigenetic regulation for miRNAs. The regions (2,500 bp upstream, 500 bp downstream of pre-miRNA) were postulated as promoters of miRNAs to investigate the epigenetic regulation of miRNA expression [25] . So we chose this region as a potential promoter to investigate the epigenetic regulation of stage-specific miRNAs during DC development and differentiation. Acetylation of histone was a general marker associated with actively transcribed promoter [26] , and acetylation of histone in the promoter regions of stage-specific miRNAs were assayed by chromatin immunoprecipitation (ChIP) assay. For miRNA expression, miR-1 and miR-486 were highly expressed in HSCs, whereas poorly expressed in other three stages; miR-132 and miR-147 were highly expressed in imDCs and maDCs, whereas poorly expressed in HSCs and DCreg; and miR-125a-5p and miR-99a were highly expressed in DCreg, whereas poorly expressed in other three stages ( Fig. 3a ). These results were confirmed by qRT–PCR assays ( Fig. 3b ), and pri-miRNA transcripts of these miRNAs were also confirmed by qRT–PCR ( Fig. 3c ). ChIP assays on the potential promoters of the above stage-specific miRNAs were analysed using two sets of qPCR primers spanning the promoters ( Fig. 3d ), and results showed that acetylation of histone H3 in the promoter regions of miR-1-1 and miR-486 were high only in HSCs; acetylation of histone H3 in the promoter regions of miR-132 and miR-147 were high only in imDCs and maDCs, whereas acetylation of histone H3 in the promoter regions of miR-99a and miR-125a were high only in DCreg ( Fig. 3e ), which were consistent with the stage-specific expression of these miRNAs. Our results suggest that stage-specific miRNAs undergo epigenetic reprogramming during cell development and differentiation. 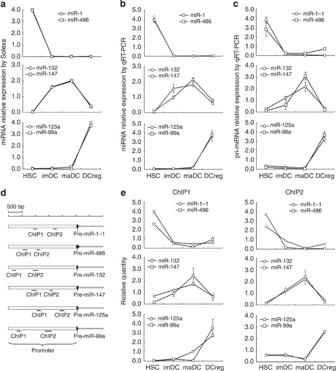Figure 3: Histone modification reprogramming in the promoter region of stage-specific miRNAs in HSCs, imDCs, maDCs and DCreg. (a) miR-132, miR-147, miR-486, miR-1, miR-99a and miR-125a-5p were detected as stage-specific miRNAs by Illumina sequencing in HSCs, imDCs, maDCs and DCreg. Data are shown as mean±s.d. (n=4) of one representative experiment. Similar results were obtained in three independent experiments. (b) miR-132, miR-147, miR-486, miR-1, miR-99a and miR-125a-5p were verified as stage-specific miRNAs by qRT–PCR in HSCs, imDCs, maDCs and DCreg. Data are shown as mean±s.d. (n=4) of one representative experiment. Similar results were obtained in three independent experiments. (c) pri-miR-132, pri-miR-147, pri-miR-486, pri-miR-1-1, pri-miR-99a and pri-miR-125a were tested by qRT–PCR in HSCs, imDCs, maDCs and DCreg. Data are shown as mean±s.d. (n=4) of one representative experiment. Similar results were obtained in three independent experiments. (d) Two sets of primers were used in the qPCR analysis to span the potential promoter of miR-132, miR-147, miR-486, miR-1-1, miR-99a and miR-125a. (e) qPCR analysis of histone H3 acetylation in the promoter region of miR-132, miR-147, miR-486, miR-1-1, miR-99a and miR-125a by ChIP assay in HSCs, imDCs, maDCs and DCreg. Data are shown as mean±s.d. (n=4) of one representative experiment. Similar results were obtained in three independent experiments. Figure 3: Histone modification reprogramming in the promoter region of stage-specific miRNAs in HSCs, imDCs, maDCs and DCreg. ( a ) miR-132, miR-147, miR-486, miR-1, miR-99a and miR-125a-5p were detected as stage-specific miRNAs by Illumina sequencing in HSCs, imDCs, maDCs and DCreg. Data are shown as mean±s.d. ( n =4) of one representative experiment. Similar results were obtained in three independent experiments. ( b ) miR-132, miR-147, miR-486, miR-1, miR-99a and miR-125a-5p were verified as stage-specific miRNAs by qRT–PCR in HSCs, imDCs, maDCs and DCreg. Data are shown as mean±s.d. ( n =4) of one representative experiment. Similar results were obtained in three independent experiments. ( c ) pri-miR-132, pri-miR-147, pri-miR-486, pri-miR-1-1, pri-miR-99a and pri-miR-125a were tested by qRT–PCR in HSCs, imDCs, maDCs and DCreg. Data are shown as mean±s.d. ( n =4) of one representative experiment. Similar results were obtained in three independent experiments. ( d ) Two sets of primers were used in the qPCR analysis to span the potential promoter of miR-132, miR-147, miR-486, miR-1-1, miR-99a and miR-125a. ( e ) qPCR analysis of histone H3 acetylation in the promoter region of miR-132, miR-147, miR-486, miR-1-1, miR-99a and miR-125a by ChIP assay in HSCs, imDCs, maDCs and DCreg. Data are shown as mean±s.d. ( n =4) of one representative experiment. Similar results were obtained in three independent experiments. Full size image Identification of new miRNA candidates We next identified new miRNA genes among the unannotated sequences in the processes of DC development and differentiation. A total of 53 new miRNA candidates were identified by ‘MIREAP’ algorithm in at least two samples of DCs in vitro ( Supplementary Table S2 ) [27] . Five novel miRNAs (DCm009, DCm015, DCm024, DCm033 and DCm044) were also confirmed to exist in the in vivo counterpart of mature DCs by Illumina sequencing. All new miRNA candidates were confirmed by qRT–PCR analysis in order to independently validate their existence, and 40 of them were validated by qRT–PCR in myelogenous cell line RAW264.7 (RAW) cells ( Fig. 4a and Supplementary Table S2 ). 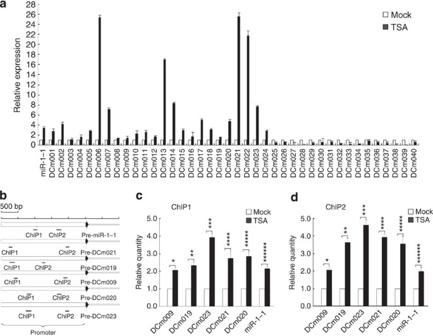Figure 4: TSA treatment increases acetylation of histone H3 and new miRNA candidate expression. (a) qRT–PCR analysis of novel miRNA candidates in RAW cells treated with DMSO or 0.5 μM TSA for 24 h. miR-1-1 was used as positive control. Data are shown as mean±s.d. (n=4) of one representative experiment. Similar results were obtained in three independent experiments. (b) Two sets of primers were used in the qPCR analysis to span the potential promoter of representative new miRNA candidates and miR-1-1. (c) qPCR analysis of histone H3 acetylation in the promoter region of representative new miRNA candidates by ChIP 1 assay in RAW cells treated with DMSO or 0.5 μM TSA. miR-1-1 was used as positive control. Data are shown as mean±s.d. (n=4) of one representative experiment. Similar results were obtained in three independent experiments. *P=0.0415, **P=0.0312, ***P=0.0023, ****P=0.0278, *****P=0.0345, *****P=0.0076 (two-tailed Student’st-test). (d) qPCR analysis of histone H3 acetylation in the promoter region of representative new miRNA candidates by ChIP 2 assay in RAW cells treated with DMSO or 0.5 μM TSA. miR-1-1 was used as positive control. Data are shown as mean±s.d. (n=4) of one representative experiment. Similar results were obtained in three independent experiments. *P=0.0275, **P=0.0167, ***P=0.0012, ****P=0.0033, *****P=0.0243, *****P=0.0279 (two-tailed Student’st-test). Figure 4: TSA treatment increases acetylation of histone H3 and new miRNA candidate expression. ( a ) qRT–PCR analysis of novel miRNA candidates in RAW cells treated with DMSO or 0.5 μM TSA for 24 h. miR-1-1 was used as positive control. Data are shown as mean±s.d. ( n =4) of one representative experiment. Similar results were obtained in three independent experiments. ( b ) Two sets of primers were used in the qPCR analysis to span the potential promoter of representative new miRNA candidates and miR-1-1. ( c ) qPCR analysis of histone H3 acetylation in the promoter region of representative new miRNA candidates by ChIP 1 assay in RAW cells treated with DMSO or 0.5 μM TSA. miR-1-1 was used as positive control. Data are shown as mean±s.d. ( n =4) of one representative experiment. Similar results were obtained in three independent experiments. * P =0.0415, ** P =0.0312, *** P =0.0023, **** P =0.0278, ***** P =0.0345, ***** P =0.0076 (two-tailed Student’s t -test). ( d ) qPCR analysis of histone H3 acetylation in the promoter region of representative new miRNA candidates by ChIP 2 assay in RAW cells treated with DMSO or 0.5 μM TSA. miR-1-1 was used as positive control. Data are shown as mean±s.d. ( n =4) of one representative experiment. Similar results were obtained in three independent experiments. * P =0.0275, ** P =0.0167, *** P =0.0012, **** P =0.0033, ***** P =0.0243, ***** P =0.0279 (two-tailed Student’s t -test). Full size image These new miRNA candidates were expressed at very low levels. To investigate whether these new miRNA candidates were silenced by epigenetic modifications, we detected the miRNA expression in RAW cells upon treatment with HDAC inhibitor Trichostatin A (TSA). A total of 24 new miRNA candidates were upregulated upon TSA treatment, and miR-1-1 was used as positive control ( Fig. 4a and Supplementary Table S2 ) [28] . ChIP assays on the potential promoter of representative candidates (DCm009, DCm019, DCm020, DCm021 and DCm023), using two sets of qPCR primers spanning the promoter ( Fig. 4b ), showed upregulation of histone H3 acetylation in TSA treatment group ( Fig. 4c,d ), miR-1-1 was used as positive control. In summary, although miRNA candidates were mainly expressed at low levels, 75% (40/53) of new miRNA candidates were detected by qRT–PCR in RAW cells. Among the qRT–PCR-positive candidates, 60% (24/40) were detected by upregulation upon TSA treatment. These new miRNA candidates may therefore represent a part of new miRNAs with unknown function. Upregulation of miR-30b in regulatory DCs by TGF-β/Smad3 Interestingly, multiple differentially expressed miRNAs were detected at different stages of DC development and differentiation, thus suggesting that many miRNAs may function in this process. We found that, compared with maDCs, miR-30b expression significantly increased in DCreg ( Fig. 5a ). As we reported previously, endothelial-like splenic stromal cells can secrete TGF-β to drive the differentiation from maDC to DCreg [15] . Therefore, we wondered whether the neutralizing antibody against TGF-β could influence miR-30b expression in DCreg. As shown in Fig. 5b , the addition of neutralizing antibody against TGF-β in the co-cultural system could decrease miR-30b expression in DCreg. Further, Smad3 deficiency decreased miR-30b expression in DCreg ( Fig. 5c ). Furthermore, as acetylation level of histone in promoter region is always elevated by Smad3 activation [29] , [30] , ChIP assays showed the upregulated histone H3 acetylation level and Smad3-binding activity in promoter region of miR-30b in DCreg compared with maDCs ( Fig. 5d–f ). To delineate whether Smad3 specifically binds miR-30b promoter in response to TGF-β, we performed silico analysis (rVista 2.0, http://rvista.dcode.org/ ) [31] to search for potential Smad-binding sites in miR-30b promoter. In this study, we found two potential Smad-binding sites in miR-30b promoter ( Fig. 5g ). To confirm this finding, we used luciferase reporter assay to determine the interaction of Smad3 with the miR-30b promoter region in RAW264.7 cells. As shown in Fig. 5h , TGF-β could successfully upregulate luciferase activity containing the potential Smad-binding sites (S1 and S2), supporting that Smad3 could physically interact with the miR-30b promoter region. These data demonstrated that upregulation of miR-30b expression in DCreg could be induced through TGF-β/Smad3-dependent pathway. 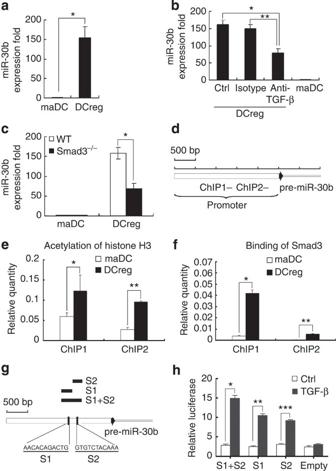Figure 5: TGF-β/Smad3-dependent pathways are responsible for the increased miR-30b expression in DCreg. (a) miR-30b expression in mouse maDCs and DCreg were detected by qRT–PCR. *P<0.0001 (two-tailed Student’st-test). Data are shown as means ±s.d. (n=3). (b) Neutralizing antibody against mouse TGF-β (5μg ml−1) or isotype antibody was added into the co-culture system between endothelial-like splenic stromal cells and maDCs. After 7 days, maDCs and DCreg were collected, and miR-30b expression was detected by qRT–PCR. Data are shown as means ±s.d. (n=3). *P=0.0014, **P=0.0021 (two-tailed Student’st-test). (c) maDCs and DCreg from wild-type or Smad3-deficient mice were collected, and miR-30b expression was detected by qRT–PCR. Data are shown as means ±s.d. (n=3). *P=0.0236 (two-tailed Student’st-test). (d) Two sets of primers were used in the qPCR analysis to span the potential promoter region of miR-30b. (e) qPCR analysis of histone H3 acetylation in the promoter region of miR-30b by ChIP assay in maDCs and DCreg. Data are shown as mean±s.d.(n=3). *P=0.0228, **P=0.0374 (two-tailed Student’st-test). (f) qPCR analysis of Smad3 binding in the promoter region of miR-30b by ChIP assay in maDCs and DCreg. Data are shown as mean±s.d. (n=4). *P=0.0153, **P=0.0286 (two-tailed Student’st-test). (g) Two predicted Smad3-binding sites (S1 and S2) were indicated in the potential promoter region of miR-30b. Three sequences including S1 or S2 sites were individually, or in combination cloned into pGL3 luciferase reporter plasmid and indicated in the potential promoter region of miR-30b. (h) Transcriptional activation from the predicted Smad3 binding sites was induced by TGF-β in RAW cells. Cells were co-transfected with luciferase reporter including Smad3-binding sites and pRL-TK. After 48 h, cells were treated with TGF-β for 4 h and luciferase values were measured. pRL-TK was co-transfected as an internal control to correct the differences in both transfection and harvest efficiencies. The firefly luciferase activity of each sample was normalized to the Renilla luciferase activity. Data are shown as mean±s.d. (n=4). Similar results were obtained in three independent experiments. *P=0.0008, **P=0.0002, ***P=0.0006 (two-tailed Student’st-test). Figure 5: TGF-β/Smad3-dependent pathways are responsible for the increased miR-30b expression in DCreg. ( a ) miR-30b expression in mouse maDCs and DCreg were detected by qRT–PCR. * P <0.0001 (two-tailed Student’s t -test). Data are shown as means ±s.d. ( n =3). ( b ) Neutralizing antibody against mouse TGF-β (5μg ml −1 ) or isotype antibody was added into the co-culture system between endothelial-like splenic stromal cells and maDCs. After 7 days, maDCs and DCreg were collected, and miR-30b expression was detected by qRT–PCR. Data are shown as means ±s.d. ( n =3). * P =0.0014, ** P =0.0021 (two-tailed Student’s t -test). ( c ) maDCs and DCreg from wild-type or Smad3-deficient mice were collected, and miR-30b expression was detected by qRT–PCR. Data are shown as means ±s.d. ( n =3). * P =0.0236 (two-tailed Student’s t -test). ( d ) Two sets of primers were used in the qPCR analysis to span the potential promoter region of miR-30b. ( e ) qPCR analysis of histone H3 acetylation in the promoter region of miR-30b by ChIP assay in maDCs and DCreg. Data are shown as mean±s.d. ( n =3). * P =0.0228, ** P =0.0374 (two-tailed Student’s t -test). ( f ) qPCR analysis of Smad3 binding in the promoter region of miR-30b by ChIP assay in maDCs and DCreg. Data are shown as mean±s.d. ( n =4). * P =0.0153, ** P =0.0286 (two-tailed Student’s t -test). ( g ) Two predicted Smad3-binding sites (S1 and S2) were indicated in the potential promoter region of miR-30b. Three sequences including S1 or S2 sites were individually, or in combination cloned into pGL3 luciferase reporter plasmid and indicated in the potential promoter region of miR-30b. ( h ) Transcriptional activation from the predicted Smad3 binding sites was induced by TGF-β in RAW cells. Cells were co-transfected with luciferase reporter including Smad3-binding sites and pRL-TK. After 48 h, cells were treated with TGF-β for 4 h and luciferase values were measured. pRL-TK was co-transfected as an internal control to correct the differences in both transfection and harvest efficiencies. The firefly luciferase activity of each sample was normalized to the Renilla luciferase activity. Data are shown as mean±s.d. ( n =4). Similar results were obtained in three independent experiments. * P =0.0008, ** P =0.0002, *** P =0.0006 (two-tailed Student’s t -test). Full size image miR-30b enhances IL-10 and NO by targeting Notch1 In order to further investigate the biological significance of the upregulated miR-30b expression in DCreg, we went further to investigate the effects of miR-30b in cytokine production of DCreg. As we reported previously [15] , [32] , IL-10 and NO were preferentially produced in DCreg, acting as important negative regulators of immune response. Further, we found that miR-30b overexpression could enhance IL-10 and NO production in DCreg, whereas miR-30b inhibition could decrease their production ( Fig. 6a ), indicating that miR-30b may contribute to the preferential IL-10 and NO production in DCreg. On a per-cell basis, similar results of IL-10 production were observed, as determined by intracellular cytokine staining ( Fig. 6b ), further indicating that miR-30b influences IL-10 production by regulatory DCs. 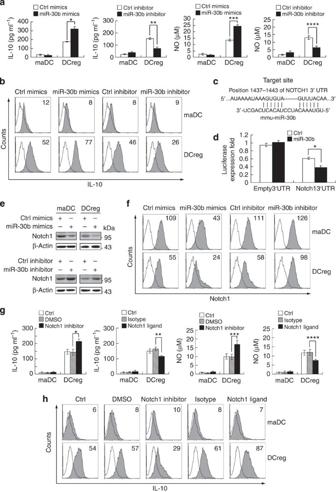Figure 6: miR-30b promotes preferential IL-10 and NO production in DCreg through targeting Notch1. (a) maDCs and DCreg (5 × 105per ml) were transfected with control mimics or miR-30b mimics, control inhibitor or miR-30b inhibitor as indicated. After 48 h, IL-10 (left) and NO (right) in supernatants was measured by ELISA and Griess assay, respectively. Data are shown as means ±s.d. (n=3). Similar results were obtained in three independent experiments. *P=0.0005, **P=0.0007, ***P=0.0004, ****P=0.0034 (two-tailed Student’st-test). (b) Flow cytometry analysis of intracellular staining for IL-10 expression of DCs transfected as in (a). Numbers in the histograms indicate the geometric mean fluorescence of the test samples. Similar results were obtained in at least three independent experiments. (c) Mouse Notch1 might be molecular target of miR-30b. Shown is a sequence alignment of miR-30b and its target sites in 3′UTR of Notch1, which was downloaded from TargetScan (http://www.targetscan.org). (d) HEK293 cells (1 × 104) were co-transfected with pGL3 firefly luciferase reporter plasmids or pGL3-Notch1 3′UTR firefly luciferase reporter plasmids, pTK–Renilla-luciferase plasmids, together with ctrl mimics or miR-30b mimics as indicated. After 24 h, firefly luciferase activity was measured and normalized by Renilla luciferase activity. Data are shown as means ±s.d. (n=3). Similar results were obtained in three independent experiments. *P=0.0033 (two-tailed Student’st-test). (e) maDCs and DCreg (1 × 106) were transfected as described in (a). After 48 h, Notch1 and β-actin were detected. (f) maDCs and DCreg were transfected with miR-30b mimics or miR-30b inhibitor as in (e). The surface expression of Notch1 expression was detected by flow cytometry. Numbers in the histograms indicate the geometric mean fluorescence of the test samples. (g) Cells were treated with mouse Delta 4 (0.5 μg ml−1) or γ-SiX (10 μM) for 18 h. IL-10 (left) and NO (right) in supernatants were measured by ELISA and Griess assay, respectively. Data are shown as means±s.d. (n=3). Similar results were obtained in three independent experiments. *P=0.0095, **P=0.0031, ***P=0.0125, ****P=0.0132 (two-tailed Student’st-test). (h) maDCs and DCreg were treated as in (g) as indicated. Expression of IL-10 was detected by intracellular staining. Numbers in the histograms indicate the geometric mean fluorescence of the test samples. Similar results were obtained in at least three independent experiments. Figure 6: miR-30b promotes preferential IL-10 and NO production in DCreg through targeting Notch1. ( a ) maDCs and DCreg (5 × 10 5 per ml) were transfected with control mimics or miR-30b mimics, control inhibitor or miR-30b inhibitor as indicated. After 48 h, IL-10 (left) and NO (right) in supernatants was measured by ELISA and Griess assay, respectively. Data are shown as means ±s.d. ( n =3). Similar results were obtained in three independent experiments. * P =0.0005, ** P =0.0007, *** P =0.0004, **** P =0.0034 (two-tailed Student’s t -test). ( b ) Flow cytometry analysis of intracellular staining for IL-10 expression of DCs transfected as in ( a ). Numbers in the histograms indicate the geometric mean fluorescence of the test samples. Similar results were obtained in at least three independent experiments. ( c ) Mouse Notch1 might be molecular target of miR-30b. Shown is a sequence alignment of miR-30b and its target sites in 3′UTR of Notch1, which was downloaded from TargetScan ( http://www.targetscan.org ). ( d ) HEK293 cells (1 × 10 4 ) were co-transfected with pGL3 firefly luciferase reporter plasmids or pGL3-Notch1 3′UTR firefly luciferase reporter plasmids, pTK–Renilla-luciferase plasmids, together with ctrl mimics or miR-30b mimics as indicated. After 24 h, firefly luciferase activity was measured and normalized by Renilla luciferase activity. Data are shown as means ±s.d. ( n =3). Similar results were obtained in three independent experiments. * P =0.0033 (two-tailed Student’s t -test). ( e ) maDCs and DCreg (1 × 10 6 ) were transfected as described in ( a ). After 48 h, Notch1 and β-actin were detected. ( f ) maDCs and DCreg were transfected with miR-30b mimics or miR-30b inhibitor as in ( e ). The surface expression of Notch1 expression was detected by flow cytometry. Numbers in the histograms indicate the geometric mean fluorescence of the test samples. ( g ) Cells were treated with mouse Delta 4 (0.5 μg ml −1 ) or γ-SiX (10 μM) for 18 h. IL-10 (left) and NO (right) in supernatants were measured by ELISA and Griess assay, respectively. Data are shown as means±s.d. ( n =3). Similar results were obtained in three independent experiments. * P =0.0095, ** P =0.0031, *** P =0.0125, **** P =0.0132 (two-tailed Student’s t -test). ( h ) maDCs and DCreg were treated as in ( g ) as indicated. Expression of IL-10 was detected by intracellular staining. Numbers in the histograms indicate the geometric mean fluorescence of the test samples. Similar results were obtained in at least three independent experiments. Full size image As miRNAs function mainly through repressing their targets, we examined the targets of miR-30b, which might modulate the preferential IL-10 and NO production in DCreg. By targets prediction of miR-30b via TargetScan ( http://www.targetscan.org ), we found that mouse Notch1 had one putative conserved miR-30b target site ( Fig. 6c ). To certify whether Notch1 was regulated post-transcriptionally by miR-30b, we constructed reporter plasmids containing the 3′UTR region of mouse Notch1, and found that its expression was significantly decreased by miR-30b co-transfection ( Fig. 6d ). Furthermore, Notch1 protein level was decreased by miR-30b overexpression, whereas elevated by miR-30b inhibition in DCs ( Fig. 6e ), confirming that miR-30b targets Notch1. Similar results were observed in flow cytometry analysis of the surface expression of Notch1 on DCs after miR30b manipulation ( Fig. 6f ), further confirming that miR-30b targets Notch1. Next, we examined the roles of Notch1 in cytokine production in DCreg, and we found that inhibition of Notch1, just like miR-30b overexpression, increased IL-10 and NO production in DCreg, and Notch1 ligand, which activates Notch1 signaling, repressed IL-10 and NO production in DCreg ( Fig. 6g ). These results further confirm the enhancing effect of Notch1 signaling on IL-10 and NO production in DCreg. Similar results of IL-10 production were observed, as determined by intracellular cytokine staining ( Fig. 6h ). Additionally, we found that the enhanced Notch1 expression was significantly downregulated by Notch1-specific small interfering RNA (siRNA) once miR-30b was inhibited. ( Fig. 7a ). Notch1-specific siRNA could rescue miR-30b inhibition-induced decrease of IL-10 and NO production in DCreg ( Fig. 7b ). Similar results of IL-10 production were also observed in the experiments with intracellular cytokine staining ( Fig. 7c ). 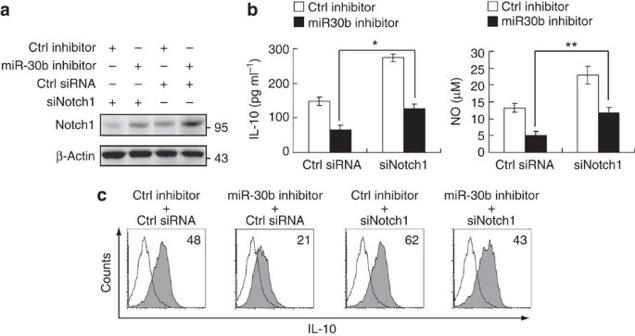Figure 7: Effect of Notch1 knockdown on preferential IL-10 and NO production in DCreg. (a) DCreg were transfected with control inhibitor or miR-30b inhibitor as in (6a). After 36 h, the cells were transfected with control small RNA (Ctrl) or Notch1-specific siRNA. After 36 h, Notch1 expression in the cells was detected. (b) DCreg were transfected as in (a). After 36 h, IL-10 (left) and NO (right) in supernatants were measured by ELISA and Griess assay, respectively. Data are shown as means ±s.d. (n=3). Similar results were obtained in three independent experiments. *P=0.0069, **P=0.0042 (two-tailed Student’st-test). (c) Flow cytometry analysis of intracellular staining for IL-10 expression of DCreg transfected as in (S2a). Numbers in the histograms indicate the geometric mean fluorescence of the test samples. Similar results were obtained in at least three independent experiments. Figure 7: Effect of Notch1 knockdown on preferential IL-10 and NO production in DCreg. ( a ) DCreg were transfected with control inhibitor or miR-30b inhibitor as in (6a). After 36 h, the cells were transfected with control small RNA (Ctrl) or Notch1-specific siRNA. After 36 h, Notch1 expression in the cells was detected. ( b ) DCreg were transfected as in ( a ). After 36 h, IL-10 (left) and NO (right) in supernatants were measured by ELISA and Griess assay, respectively. Data are shown as means ±s.d. ( n =3). Similar results were obtained in three independent experiments. * P =0.0069, ** P =0.0042 (two-tailed Student’s t -test). ( c ) Flow cytometry analysis of intracellular staining for IL-10 expression of DCreg transfected as in (S2a). Numbers in the histograms indicate the geometric mean fluorescence of the test samples. Similar results were obtained in at least three independent experiments. Full size image miRNAs have been shown to regulate mammalian immune cell differentiation, development and influence the outcome of immune responses, and also they are spatially and temporally regulated in a panel of mammalian tissues and cell types [33] . Whereas DCs are of vital importance in linking innate and adaptive immune responses, the function of intrinsic miRNAs in DCs remains elusive. In order to elucidate the alteration of individual miRNA, several methods, including qRT–PCR [34] and microarray [35] techniques have been widely used in qualitative miRNA studies. However, these approaches have low throughput with low sensitivity and poor resolution, which lack vigor in revealing the abundance of each miRNA in the background of the entire miRNome. At present, MPSS of miRNAs can identify the entire miRNome in-depth and explore miRNA expression differences as well as the individual miRNA abundance in a given tissue or cell type under a certain physiological or pathological context. We have carried out Illumina sequencing analysis to define the miRNomes in human liver and hepatocellular carcinoma [36] and also in human NK cells [10] , revealing the miRNA candidates involved. To date, Illumina sequencing analysis of the miRNomes in mouse bone marrow HSCs and DCs at different differentiation stages remains to be performed. The Illumina sequencing used in this study led to the identification of a large fraction of miRNA expressed during DC development and differentiation in vitro and in vivo . These included 53 new miRNA candidates, as well as a potentially distinct class of short RNAs not fulfilling current criteria for miRNAs. These findings have general implications for the understanding of the total miRNA content of the mouse genome as well as for future studies on the role of miRNAs in DC development, differentiation and function, and also in stem cell biology. Although most miRNAs are known and most of them are ubiquitously expressed [37] , additional analyses of purified cell populations have partially identified the existence of tissue- and stage-specific miRNAs in a few tissues. Illumina sequencing analysis of miRNome has viewed of expressed miRNAs over a wide dynamic range of expression levels in several kinds of tissues and cell types such as human embryonic stem cells, human B cells and mouse NK cells [20] , [38] , [39] . However, the full scale of miRNomes in various DC subsets and HSCs remains to be fully identified. In the present study, the miRNomes of DC development and differentiation in vitro and in vivo , including HSCs, imDCs, maDCs and DCreg have been revealed. Our results reveal that, during DC development and differentiation, miRNA expression spectrums were similar, but miRNA expression profiles changed significantly, especially in DC development and differentiation processes. The miRNAs, preferentially expressed at one or two stages, may raise interesting future work to elucidate the detailed roles of these miRNAs in the regulation of DC development and differentiation. Epigenetic modification involved in the regulation of gene expression has been widely investigated, mainly focusing on protein-coding genes. Many of these genes with tissue-specific expression undergo epigenetic reprogramming during cell development and differentiation [40] , [41] . However, epigenetic regulation of non-protein-coding genes, especially miRNAs, is not yet clear. As reported, some tissue or stage-specific miRNAs are regulated by epigenetic modification in their promoter regions [42] , [43] , [44] , such as the low miR-1-1 expression in hepatocellular carcinoma was due to DNA methylation and histone deacetylation in its promoter region [28] . Therefore, we explored the possibility that whether stage-specific miRNAs were regulated by epigenetic modification in their promoter during DC development and differentiation. In the processes of DC development and differentiation, many miRNAs demonstrated stage-specific expression, and we have demonstrated that some of them were regulated by histone acetylation. However, as DNA methylation and histone methylation are also important epigenetic modifications in regulating gene expression, an interesting topic that remains to be investigated is whether the differentially expressed miRNAs in DC development and differentiation are also mediated by these epigenetic modifications. miRNAs are spatially and temporally expressed in multiple types of immune cells, suggesting their specific roles in the development and function of these immune cells. Based on analysis of miRNomes, we went further to find that, compared with maDCs, miR-30b expression was significantly enriched in DCreg in vitro and in vivo . We further investigated the underlying mechanism for the miR-30b enrichment in DCreg. In our previous report, endothelial-like splenic stromal cells can induce the differentiation from maDCs to DCreg, which is dependent on TGF-β production [15] . TGF-β is a pleiotropic growth factor that modulates immune response by controlling cell proliferation, cell differentiation and apoptosis. Upon activation, TGF-β activates Smad3, which subsequently translocates into the nucleus and initiates transcription of target genes. Despite the known roles of TGF-β/Smad3 signaling in regulating immune response, such as modulation of cytokine production, its roles in regulating miRNA expression remain unknown. Here we showed that the enriched expression of miR-30b in DCreg was dependent on TGF-β/Smad3 signaling, and more Smad3 binding to the acetylated promoter region of miR-30b in DCreg. These data have suggested a new model of gene expression regulation mediated by activated TGF-β/Smad3 signaling, which may present indications in researching the mechanisms of TGF-β regulating immune response. In the immune system, Notch signaling, as a highly conserved pathway, has been implicated in determining cell fate including cell growth, differentiation and survival. Recently, the role of Notch signaling has been found to be important in the function of antigen-presenting cells [45] . Our work showed that Notch1 and downstream signaling, targeted by the enriched miR-30b expression in DCreg, negatively regulated the preferential IL-10 and NO production in DCreg, which is consistent with the recent report that Notch1 signaling could inhibit IL-10 production in macrophages stimulated with TLR agonists [46] . More recently, we demonstrated that Notch signaling suppressed TLR-triggered inflammatory cytokine production by inhibiting ERK1/2-mediated NF-κB activity in macrophages [47] . We previously found that upregulated IL-10 production might be due to enhanced activation of ERK1/2 in DCreg [48] . Our findings suggest that miR-30b can target Notch1 to retain the negative regulatory role of DCreg through enhanced activation of ERK1/2. In contrast, previous reports presented that Notch signaling was required for IL-10 production in T cells [49] . These discrepancies may be due to the distinct roles of Notch1 signaling in the different cell types, which may include the different epigenetic modification in the promoters of IL-10 and NO or the different activation of multiple transcription factors to the binding sites of IL-10 and NO promoter regions, thus suggesting distinct regulatory mechanisms in different cell types. In summary, through Illumina sequencing, we present a more comprehensive understanding of the miRNomes during DC development and differentiation. miRNA expression profiles change significantly, especially at the developmental stage from HSCs to imDCs as well as the differentiational stage from maDCs to DCreg, while they are relative stable during the DC maturation process. Many stage-specific miRNAs undergo epigenetic reprogramming in their promoter regions, suggesting their specific functions in specific stages. Among them, miR-30b is an enriched miRNA in DCreg, which contributes to the preferential IL-10 and NO production in diffDCs through targeting Notch1. Our results provide a resource for researching the roles of miRNAs in DC development, differentiation and function. In addition, miRNome of mouse bone marrow HSCs may also provide clues for the future study of stem cell biology. Mice and reagents C57BL/6J mice at 5–6 weeks of age were obtained form Joint Ventures Sipper BK Experimental Animal Company (Shanghai, China). All animal experiments were undertaken in accordance with the National Institute of Health Guide for the Care and Use of Laboratory Animals, with the approval of the Scientific Investigation Board of Second Military Medical University, Shanghai. Recombinant mouse GM-CSF, IL-4, LPS ( Escherichia coli , O26:B6) and Delta 4 were from Sigma (St Louis, MO, USA). All primers were supplied by Sangon (Shanghai, China). Antibody against Notch1 (D1E11) was from Cell Signaling Technology (Danvers, MA, USA), antibodies against β-actin and their respective horseradish peroxidase-coupled secondary antibodies were from Santa Cruz (Santa Cruz, CA, USA), antibodies against Lineage(Lin), c-Kit and Scal were from eBioscience (San Diego, CA, USA). γ-secretase inhibitor X (γ-SiX) was from Calbiochem (San Diego, CA, USA). Preparation of bone marrow-derived DC subsets Mouse imDCs were prepared from bone marrow progenitors by culturing in 10 ng ml −1 rmGM-CSF and 1 ng ml −1 rmIL-4. Nonadherent cells were gently washed out on the third day of culture; the remaining loosely adherent clusters were used on day 6 as imDCs. DCreg derived from maDCs were generated by co-culturing with splenic stroma [15] . Sorting of HSCs and natural counterparts of DCs in vivo To purify HSCs, bone-marrow cells were stained with antibodies and Lin − c-Kit + Sca1 + population was sorted using a MoFlo XDP cell sorter (Beckman Coulter), and the purity was confirmed to be >95%. CD11c + cells enriched by CD11c-conjugated microbeads from spleen were stained with fluorescently labeled anti-Ia-FITC, and then CD11c + Ia low cells and CD11c + Ia high cells were sorted using a MoFlo XDP cell sorter (Beckman Coulter) [15] . Small RNA library preparation and Illumina sequencing Total RNA of HSCs and bone marrow-derived DC subsets was isolated using mirVana miRNA Isolation Kit (Ambion) according to the manufacturer’s instructions. After PAGE purification of small RNA molecules under 30 bases and ligation of a pair of adaptors to their 5′ and 3′ ends, the small RNA molecules were amplified and sequenced on an Illumina platform according to the manufacturer’s instructions [36] . Small RNA annotation Small RNA sequences were analysed and annotated. We performed database search to assign each small RNA sequence a unique annotation and classify small RNAs into different categories according to their annotations. Unique small RNA sequences were mapped to reference sequences by SOAP ( http://soap.genomics.org.cn ). We mapped small RNAs to genomic sequences by blast, blast small RNAs against these known non-coding RNAs such as rRNA, tRNA, snRNA and snoRNA which deposited at Rfam database then annotated these small RNAs as ‘rRNA etc.’ With the repeat annotations of the reference genome available, by a parallel overlap finding algorithm, small RNAs positioned at repeat loci are identified. Using a parallel overlap finding algorithm, small RNAs derived from gene regions also are separated. Small RNAs perfectly matching miRBase precursor sequence were identified as known miRNA. The remained small RNAs were classified as unannotated. Identification of novel miRNA candidates After the annotation of known miRNAs, the remaining sequences were aligned to mouse genome to predict novel miRNA candidates. Bioinformatic prediction of novel miRNA candidates was based on the characteristics of miRNAs, which are 18–25 nucleotides in length and processed from their hairpin-like precursors with characteristic fold-back structure using ‘MIREAP’ ( https://sourceforge.net/projects/mireap/ ) [27] . RNA quantification Real-time qRT–PCR assay was performed to measure the expression of miRNA using stem-loop RT primer and expression of pri-miRNA using oligo(dT) RT primer. Expressions of miRNA and pri-miRNA were normalized to the expression of U6 and β-actin in each sample, respectively. All primers were listed in Supplementary Data 3 . ChIP assay The cells were crosslinked and processed according to the UpState Chromatin Immunoprecipitation (ChIP) Assay Kit protocol (UpState 17–295). Antibodies to acetyl-Histone H3 (Millipore 06–599), Smad3 (Cell Signaling 9523) and control IgG (Santa Cruz sc-2027) were used at 5 μg per immunoprecipitation. Ten microlitres of sonicated but pre-immunoprecipitated DNA from each sample was used as input control. ChIP results were analysed by real-time PCR. All results were normalized to input in each sample. All primers were listed in Supplementary Data 3 . Assays for IL-10 and NO IL-10 in the culture supernatants collected at the indicated times were assayed by using ELISA kits (R&D Systems). NO production was assayed by measurement of the nitrite concentration with the Griess assay [15] . Immunoblot Cells were lysed using M-PER Protein Extraction Reagent (Pierce, Rockford, IL, USA) supplemented with protease inhibitor cocktail (Calbiochem). Protein concentrations of the extracts were measured with BCA assay (Pierce) and equalized with the extraction reagent. Equal amount of the extracts were loaded and subjected to SDS–PAGE, transferred onto nitrocellulose membranes. The membrane was then incubated in a 1:1,000 dilution of a primary antibody in 5% BSA-TBS-T. After three washes in TBS-T, the membrane was incubated with 1:5,000 dilution of the corresponding secondary antibody in 5% non-fat dry milk-TBS-T and respective proteins were then blotted. [36] . Luciferase assays The Notch1 3′UTR luciferase reporter construct was prepared by amplifying the mouse Notch1 mRNA 3′UTR sequence by PCR and cloned into pMIR-Report construct (Ambion, Austin, TX, USA). Three sequences including S1 or S2 sites were individually or in combination cloned into pGL3 luciferase reporter plasmid (Promega). HEK293 cells described above were co-transfected with 80 ng luciferase reporter plasmid, 40 ng pRL–TK–Renilla-luciferase plasmid, and indicated RNAs (final concentration: 20 nM). After 24 h, Luciferase activities were measured using Dual-Luciferase Reporter Assay System (Promega) according to the man’ and in Dulbecco’s modified Eagle’s medium (DMEM ufacturer’s instructions. Data was normalized for transfection efficiency by dividing Firefly luciferase activity with that of Renilla luciferase. All primers are listed in Supplementary Data 3 . Cell culture and transfection HEK293 cell line was obtained from American Type Culture Collection (ATCC, Manassas, VA, USA) and cultured in Dulbecco’s modified Eagle’s medium (DMEM) containing 10% fetal bovine serum. The cells (1 × 10 4 ) were seeded into 96-well plates and incubated overnight. JetSI-ENDO transfection reagents (Polyplus-transfection, Illkirch, France) were used for the co-transfection of plasmids and RNAs according to the manufacturer’s instructions. Around 2 × 10 5 maDCs and DCreg were seeded into each well of 24-well plates and incubated overnight, and then transfected with RNAs using INTERFERin (Polyplus-transfection) according to the manufacturer’s instructions. miRNA mimics and inhibitors miR-30b mimics (double-stranded RNA oligonucleotides) and miR-30b inhibitors (single-stranded chemically modified oligonucleotides) from Ribobio Co. (Guangzhou, China) were used for the overexpression and inhibition of miR-30b activity in cells. Cells described above were transfected with RNAs at a final concentration of 20 nM. Negative control mimics or inhibitors (Ribobio Co.) were transfected as matched controls. Cell culture and TSA treatment Mouse myelogenous cell line RAW 264.7 cells were obtained from ATCC. RAW cells were cultured in Dulbecco’s modified Eagle’s medium (DMEM) containing 10% fetal bovine serum. Exponentially growing cells were treated with 500 nM TSA and DMSO for 24 h. The cells were harvested for RNA isolation, total RNA were subjected to qRT–PCR analysis. Statistical analysis Statistical significance was determined by Student’s t -test, with P -values of <0.05 considered to be statistically significant. Accession codes: The Illumina sequencing data has been deposited in Gene Expression Omnibus under accession numbers GSE45882 and GSE51574 . How to cite this article: Su, X. et al. miRNomes of haematopoietic stem cells and dendritic cells identify miR-30b as a regulator of Notch1. Nat. Commun. 4:2903 doi: 10.1038/ncomms3903 (2013).